Detecting noise with shot noise using on-chip photon detector The high-frequency radiation emitted by a quantum conductor presents a rising interest in quantum physics and condensed matter. However, its detection with microwave circuits is challenging. Here, we propose to use the photon-assisted shot noise for on-chip radiation detection. It is based on the low-frequency current noise generated by the partitioning of photon-excited electrons and holes, which are scattered inside the conductor. For a given electromagnetic coupling to the radiation, the photon-assisted shot noise response is shown to be independent on the nature and geometry of the quantum conductor used for the detection, up to a Fano factor, characterizing the type of scattering mechanism. Ordered in temperature or frequency range, from few tens of mK or GHz to several hundred of K or THz respectively, a wide variety of conductors can be used like Quantum Point Contacts (this work), diffusive metallic or semi-conducting films, graphene, carbon nanotubes and even molecule, opening new experimental opportunities in quantum physics. Using quantum conductors to detect high-frequency radiations is very promising [1] , [2] , [3] , [4] , [5] . However, it faces some fundamental issues. In particular, the important mismatch between the quantum conductor impedance (~ h / e 2 ) and the circuit impedance (typically 50 Ω) strongly limits the sensitivity. Recent realizations of on-chip quantum detection [6] , [7] , [8] , [9] , [10] , [11] , [12] have circumvented this issue using spatially close detectors with larger impedance providing high sensitivity up to high frequency. On-chip detectors have been realized using GaAs/AlGaAs two-dimensional electron gas (2DEG)-patterned quantum dots [8] , [9] and Aluminium or Niobium SIS junctions [6] , [10] , [12] . The photon response of quantum dots depends on an energy scale set by their geometry, and that of superconducting junctions is limited by a characteristic energy gap and both systems show tunnel resistance variability. Regarding bolometric detectors their efficiency depends on the phonon relaxation time, requires low temperature and shows slow response time. In this letter, we propose an on-chip radiation detection based on photo-assisted shot noise (PASN). When a quantum conductor is subjected to a time-dependent drain-source voltage, electrons and holes are created which then scatter inside the conductor [13] , [14] , [15] , [16] . Their partitioning between source and drain contacts leads to a current noise called PASN. Remarkably, there is a simple link between PASN and the incident radiation power up to a noise Fano factor characterizing the statistics of partitioning. This simple link is better understood if we remark that PASN is the quantum manifestation of the rectification property of ordinary shot noise [17] , [18] , [19] , [20] , which is proportional to the absolute value of the drain-source voltage. 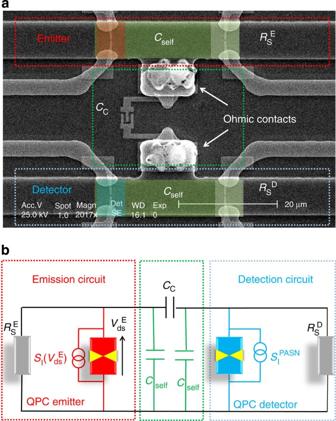Figure 1: Device structure. (a) Scanning electron microscope view of the sample. The scale bar represents a 20 μm length. Two independent circuit lines defined by wet-chemical etching of the 2DEG are coupled via the capacitanceCC. On the upper line are patterned two QPCs in series: the QPC emitter (in red), and the QPC series resistor (in white) tuned on a plateau. On the lower line, the QPC detector is coloured in blue. (b) Equivalent circuit. In red, the emitter line is coupled via the coupling capacitanceCCto the detector line in blue. The self capacitancesCselfhave been added that model the capacitance of each line between the two QPCs to the ground. Photon detection principle Figure 1 shows the principle of the on-chip detection. It consists of two separate excitation and measurement circuit lines etched in a high-mobility 2DEG. Each line involves two quantum point contacts (QPCs) in series. On the upper line, the left QPC is the high-frequency emitter. When biased by the dc voltage , it generates shot noise up to the frequency (refs 19 , 21 ). The right QPC tuned on a conductance plateau acts as a stable series resistance converting current noise into voltage noise. In the lower line, the left QPC is the detector. In series with the right QPC, also tuned on a resistance plateau , it experiences the emitter line voltage fluctuations via the coupling capacitance C C up to the cutoff frequency f max (ref. 22 ; Supplementary Fig. 1 ). The number of electron-hole pairs generated in the detector line is a direct function of the radiated noise power integrated up to frequency ( Supplementary Discussion 1 and Supplementary Fig. 2 ). Their scattering by the QPC detector generates a low-frequency PASN, which is measured. f max depends on all QPC resistances and on the self-capacitance C self of the 2DEG part between the QPCs in series. Figure 1: Device structure. ( a ) Scanning electron microscope view of the sample. The scale bar represents a 20 μm length. Two independent circuit lines defined by wet-chemical etching of the 2DEG are coupled via the capacitance C C . On the upper line are patterned two QPCs in series: the QPC emitter (in red), and the QPC series resistor (in white) tuned on a plateau. On the lower line, the QPC detector is coloured in blue. ( b ) Equivalent circuit. In red, the emitter line is coupled via the coupling capacitance C C to the detector line in blue. The self capacitances C self have been added that model the capacitance of each line between the two QPCs to the ground. Full size image To understand the photon detection principle, let us first assume that the detector line is excited by a coherent radiation at frequency Ω/2 π such that . Electrons in the detector line can absorb l photons of energy E l = lħ Ω by creating an electron-hole pair with a probability P ( E l )=| J l ( eV ac / ħ Ω)| 2 , with J l the l th Bessel function. Electrons and holes are independently and randomly partitioned by the QPC detector between left and right contacts. This generates a PASN whose low-frequency spectral density of current fluctuations is given by [13] , [14] , [15] , [16] : with T e the electronic temperature and D D, n the transmission of the n th electronic mode contributing to the QPC detector conductance G D , n =1, 2,.... We introduce the Fano factor F defined as F =∑ n D D, n (1− D D, n )/∑ n D D, n . For weak ac voltage eV ac ≪ ħ Ω and zero temperature, a direct relation can be established between the radiation power and the current noise: , where Z rad is the radiation impedance assumed smaller than the QPC detector conductance G D and F the Fano factor. In equation (1), the sum over the energies E l gives the probability to generate electron-hole pairs. This probability only depends on the excitation and not on the details of the detector. From equation (1), it is clear that the maximum PASN will be obtained for total transmission D D =∑ n D D, n = k +1/2, k an integer. In addition to shot noise, a photon-assisted dc current I ph is generated when considering the (weak) energy dependence of the QPC transmission: f (ε) is the equilibrium Fermi distribution. Photocurrent requires the energy dependence of the QPC. After photons absorption, electron-hole pairs are generated. As electrons and holes do not have the same transmission, a net DC current is induced. The energy dependence of transmission is strongly sample dependent and makes the photocurrent response not universal. On the contrary, the PASN response only depends on the Fano factor, which can be measured from conductance for a single-mode QPC, or is even universal, that is, 1/3, for a diffusive conductor. Modelling the QPC transmission with a saddle point potential [23] , [24] , it can be shown that : maximum photocurrents will be also obtained at half-integer D D . In the present case, the excitation is not coherent but due to random fluctuations of the QPC detector drain-source voltage that originates from the capacitive coupling with the noisy QPC emitter. The above expressions can be generalized, giving the PASN as: and the photocurrent: The generalized probability distribution P ( E ) is similar to the P ( E ) function used in the dynamical Coulomb blockade theory ( Supplementary Discussion 2 ). It is a direct function of the radiation power to be detected, which as a shot noise itself is maximum for D E =0.5. Photocurrent measurement We first focus on the photocurrent whose measurement set-up is described in Fig. 2a . Source V in leads to a current in the upper line and to the voltage difference across the emitter. The resulting shot noise induces a photocurrent I ph in the detector. We modulate V in at frequency 174 Hz and detect the induced photocurrent using lock-in techniques. Series resistances are tuned on a plateau for each line, whereas the emitter and detector transmissions are varied. Following the saddle point potential model of a QPC [23] , [24] , the transmission of the n th mode can be written , where V g, n is related to the negative curvature of the saddle point potential. 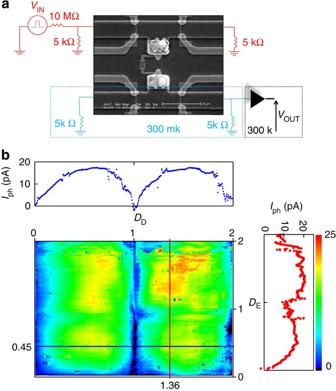Figure 2: Photocurrent measurement. (a) Schematic representation of the experimental set-up for the photocurrent measurement. The scale bar represents a 20 μm length. The QPC emitter is excited by a sine wave functionVpp~460 μV at 174 Hz. Resistances of 5 kΩ are used as current to voltage converters. By measuring the output voltageVoutafter the amplifier (black triangle in the figure), with the excitation source as a reference signal, we can extract the photocurrent. (b) The photocurrent as a function of the total transmissionsDD(xaxis) andDE(yaxis). On the upper graph is represented the photocurrent as a function ofDD(DEtuned to 0.45). The right graph shows the photocurrent as a function ofDE(DDtuned to 1.36). The photocurrent is given by ( Supplementary Discussion 3 ): Figure 2: Photocurrent measurement. ( a ) Schematic representation of the experimental set-up for the photocurrent measurement. The scale bar represents a 20 μm length. The QPC emitter is excited by a sine wave function V pp ~460 μV at 174 Hz. Resistances of 5 kΩ are used as current to voltage converters. By measuring the output voltage V out after the amplifier (black triangle in the figure), with the excitation source as a reference signal, we can extract the photocurrent. ( b ) The photocurrent as a function of the total transmissions D D ( x axis) and D E ( y axis). On the upper graph is represented the photocurrent as a function of D D ( D E tuned to 0.45). The right graph shows the photocurrent as a function of D E ( D D tuned to 1.36). Full size image V g,n and the lever arm Δ=∂ε/∂ V g are extracted from a study of the differential QPC conductance versus gate and bias voltages. We have introduced as the effective noise temperature of the circuit, which, up to a coupling factor, includes a combination of the shot noise temperature of the emitter: plus other equilibrium thermal noise contributions of the circuit surrounding the detector QPC. The coupling capacitance C C appears in via the transimpedance of the system, which characterizes the strength of the coupling. Considering the geometry of C C , independent simulations give C C ~1 fF. The colour plot in Fig. 2b shows the measured photocurrent as a function of the emitter and detector transmissions D E and D D , up to two transmitting orbital electronic modes. Above the colour plot, the photocurrent is plotted as a function of D D for a fixed value of D E ~0.45. As expected, it is maximum for half transmission of the emitter electronic modes and vanishes for integer transmission. These measurements have been found essential for a fine calibration of the electrical circuit and for complementary characterization of the PASN effect ( Supplementary Fig. 3 ). PASN detection We now consider PASN measurements. The cross-correlation noise measurement set-up is described in Fig. 3a . To characterize the detector line, the QPC detector transmission is set to D D =0.17, whereas a dc bias is applied on the detector line. The resulting shot noise measured, black dots in Fig. 3b , perfectly agrees with the theory in red solid line. We extract an electronic temperature T e =310 mK close to the fridge temperature T =300 mK. Then, we turn off the applied bias on the detector line and the QPC emitter is biased and also tuned at transmission D E =0.5. Both series resistances are tuned on the first plateau. Because of the coupling capacitance, voltage fluctuations are reported on the detector line. The only dc current flowing through the detector line being the weak dc photocurrent, no detectable transport shot noise is expected. However, we detect some noise, confirming that the PASN detection works as illustrated in Fig. 3c , black circle. 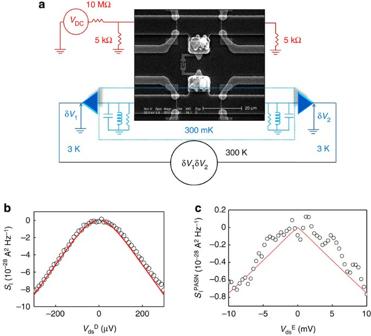Figure 3: PASN measurement. (a) Schematic representation of the experimental set-up for the PASN measurement. The QPC emitter being biased emits shot noise. Because of the capacitive coupling between the emitter and detector line, high-frequency voltage fluctuations are transferred in the detector line, generating PASN. Shot noise measurements are done by converting the current fluctuations into the voltage fluctuations (notedδV1andδV2) across a parrallel inductor-capacitor resonant circuit (RLC circuit), cooled at 300 mK using 3 MHz resonant frequency and 300 kHz typical bandwidth. Homemade cryogenic amplifiers, with ultra-low input voltage noise () and located on the 3 K stage, amplify the voltage fluctuations. Using fast acquisition card and Fast Fourier Transform, the voltage noise cross-correlation ‹δV1δV2› is computed in real time. Then ‹δV1δV2› is converted into a current shot noiseSI. (b) Measured excess shot noiseSI(thermal noise being subtracted) as a function of dc voltageacross the QPC detector, when the QPC series resistor is opened and the transmission is tuned to 0.17. (c) Measured PASNas function of theaccross the QPC emitter. QPC emitter and detector are tuned atDD=DE=0.5. Both series resistances are tuned on the first plateau. The detected PASN, , is expected to be ( Supplementary Discussion 4 ): Figure 3: PASN measurement. ( a ) Schematic representation of the experimental set-up for the PASN measurement. The QPC emitter being biased emits shot noise. Because of the capacitive coupling between the emitter and detector line, high-frequency voltage fluctuations are transferred in the detector line, generating PASN. Shot noise measurements are done by converting the current fluctuations into the voltage fluctuations (noted δV 1 and δV 2 ) across a parrallel inductor-capacitor resonant circuit (RLC circuit), cooled at 300 mK using 3 MHz resonant frequency and 300 kHz typical bandwidth. Homemade cryogenic amplifiers, with ultra-low input voltage noise ( ) and located on the 3 K stage, amplify the voltage fluctuations. Using fast acquisition card and Fast Fourier Transform, the voltage noise cross-correlation ‹ δV 1 δV 2 › is computed in real time. Then ‹ δV 1 δV 2 › is converted into a current shot noise S I . ( b ) Measured excess shot noise S I (thermal noise being subtracted) as a function of dc voltage across the QPC detector, when the QPC series resistor is opened and the transmission is tuned to 0.17. ( c ) Measured PASN as function of the accross the QPC emitter. QPC emitter and detector are tuned at D D = D E =0.5. Both series resistances are tuned on the first plateau. Full size image Here, considering P ( E ) takes only important values for E ≪ k B T e , a low-energy expansion of equation (3) has been made. The amplitude compatible with the detector geometry (estimated C self =3 fF and C C =0.9 fF) and obtained from photocurrent measurements can now be compared with the noise measurement. The theoretical prediction (red solid line) following equation (6) also includes an additional term because of heating effect. We discuss this point in the following. We open the series QPC of the detector line such that the current-to-voltage fluctuation conversion is now mediated by the smaller resistance of the long resistive mesa. Then we apply a fixed bias and sweep the detector transmission (red circles in Fig. 4a ). As expected, the shot noise is maximum for D D =0.5 and cancels for D D =1. The slight disagreement with the theoretical prediction (red solid line) around D D ~0.7 reveals a weak ‘0.7’ anomaly [25] , [26] , [27] , [28] . Then we tune the series QPC on its first plateau and repeat the same experiment (black circles). Surprisingly, the shot noise does not cancel anymore for D D =1. To understand it, we must consider heating effects ( Supplementary Discussion 5 ). As the size of the QPC is much smaller than the electron-phonon relaxation length, there is a temperature gradient from the QPC to the ohmic contacts assumed to be at the base temperature of the fridge. Combining Joule heating together with the Wiedemann–Franz law, we obtain [17] ( Supplementary Fig. 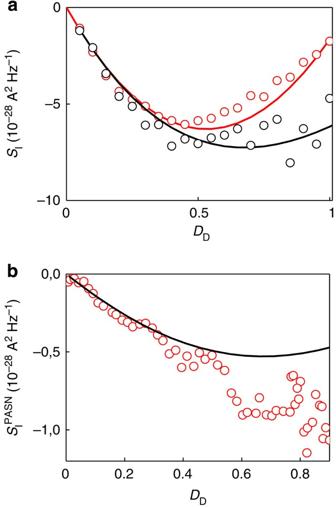Figure 4: Transmission dependence of the PASN. (a) Red dots: measured shot noise as a function ofDDfor an opened series QPC together with our theoretical model (red solid line). Black dots: same measurement with the series QPC tuned on a plateau. The non-zero value of tefhe noise forDD=1 results from heating effect. In both cases,. The noise due to the heating of the series resistance has been subtracted. (b) Red dots: measured PASN as function ofDDfor the series QPC tuned on the first plateau and a fixedDE~0.5 (theoretical prediction represented by a black solid line). The applied DC bias is. 4 ): Figure 4: Transmission dependence of the PASN. ( a ) Red dots: measured shot noise as a function of D D for an opened series QPC together with our theoretical model (red solid line). Black dots: same measurement with the series QPC tuned on a plateau. The non-zero value of tefhe noise for D D =1 results from heating effect. In both cases, . The noise due to the heating of the series resistance has been subtracted. ( b ) Red dots: measured PASN as function of D D for the series QPC tuned on the first plateau and a fixed D E ~0.5 (theoretical prediction represented by a black solid line). The applied DC bias is . Full size image with G m the total conductance linking the QPC to the ohmic contacts and T fridge the base temperature. Considering this effect, a QPC tuned on a plateau will not be noiseless anymore. We find a good agreement with measurements, black solid line. We now apply on the emitter line, fixing D E ~0.5 to get the maximum emitted signal. In Fig. 4b , the PASN is measured as a function of D D . The non-zero value of the shot noise for D D =1 results from the similar heating effect ( Supplementary Fig. 5 ). The agreement between theory and experimental data confirms our good understanding of the ‘on-chip’ detection mechanism: both photocurrent and PASN result from the same photon-assisted effect . As the photon current detector is based on the energy dependence of the transmission, which is strongly geometry dependent, it raises the question of the use of such a detector based on a common calibration. On the contrary, PASN detection only depends on the transmission. For metallic diffusive system, the Fano factor is even constant 1/3 (ref. 29 ) and such a detector could be used on a large scale. Regarding the photodetection efficiency, there is a competition between the direct coupling C C of the two lines and the shortcut to the ground characterized by C self . In the future, we will increase the number of fingers of the interdigitated C C and reduce the area between the QPC to lower C self , and therefore reach the most efficient regime where . To conclude, we have described a way of detecting high-frequency voltage fluctuations based on PASN measurement and seconded by photocurrent measurement. If the latter depends on the details of the mesoscopic conductor used, PASN is universal up to a noise Fano factor. The PASN approach for noise or photon radiation detection can be applied to other systems. This technique offers the possibility to probe mesoscopic properties at very high frequency (GHz and THz) of various materials (GaAs, graphene, carbon nanotube). Emitter and detector lines were patterned using e-beam lithography on a high-mobility 2DEG formed at the GaAs/ Ga x Al 1−x As heterojunction. The 2DEG, located at a depth of 100 nm below the surface, has a density of 1.8 × 10 11 cm −2 and mobility of 2.69 × 10 6 cm 2 V −1 s −1 . Measurements were performed in cryogen-free 3 He cryostat at 300 mK (base temperature). How to cite this article : Jompol, Y. et al . Detecting noise with shot noise using on-chip photon detector. Nat. Commun. 6:6130 doi: 10.1038/ncomms7130 (2015).